All WSe21T1R resistive RAM cell for future monolithic 3D embedded memory integration 3D monolithic integration of logic and memory has been the most sought after solution to surpass the Von Neumann bottleneck, for which a low-temperature processed material system becomes inevitable. Two-dimensional materials, with their excellent electrical properties and low thermal budget are potential candidates. Here, we demonstrate a low-temperature hybrid co-integration of one-transistor-one-resistor memory cell, comprising a surface functionalized 2D WSe 2 p- FET, with a solution-processed WSe 2 Resistive Random Access Memory. The employed plasma oxidation technique results in a low Schottky barrier height of 25 meV with a mobility of 230 cm 2 V −1 s −1 , leading to a 100x performance enhanced WSe 2 p -FET, while the defective WSe 2 Resistive Random Access Memory exhibits a switching energy of 2.6 pJ per bit. Furthermore, guided by our device-circuit modelling, we propose vertically stacked channel FETs for high-density sub-0.01 μm 2 memory cells, offering a new beyond-Si solution to enable 3-D embedded memories for future computing systems. Emerging non-von Neumann architectures with intensive in-memory computing like next-generation deep learning and neuromorphic chips will demand high-density integration of embedded memory. Three-dimensional monolithic (sequential) multilayer stacking of transistors and memory among interconnects may allow us to expand the on-chip memory density. Such architectures will not only overcome the two-dimensional (2D) die limitations but also enable new three-dimensional (3D) computation systems, where logic and memory elements are intimately co-located, to significantly improve the memory access bandwidth and energy [1] . However, to fully realize such 3D systems, there are fundamental technology challenges to overcome. Among which, transistor-interconnect thermal budget incompatibility poses a major road block. Advanced low-resistivity copper interconnect with low- k dielectric interlayer cannot tolerate thermal exposure above 400 °C [2] . Since the thermal activation of dopants in Si-based devices are typically between 600 and 1000 °C, Si transistor formation below such temperature results in device performance and reliability degradations [3] . This low thermal budget technology barrier calls for both material and process integration breakthroughs, to enable new platforms for 3D integration. Carbon nanotubes (CNTs) field-effect transistor (FETs) and 2D semiconducting van der Waal-layered crystals (2DMat) have drawn immense attention as transistor channel material, due to their intrinsic performance that rivals silicon, as well as upcoming successors like germanium, silicon germanium, and III–V compound semiconductors at sub-nanometer channel thickness regime [4] . 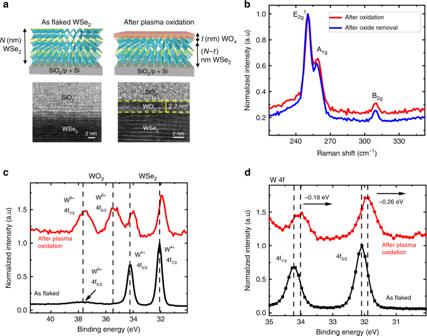Fig. 1 Remote plasma oxidation process and characterization.aSchematic representation of surface plasma oxidation and the corresponding cross-sectional transmission electron microscope (xTEM) images. The xTEM image of oxidized WSe2shows 2.2 nm of WO3upon oxidation, which is a consumption of three layers of WSe2.bRaman spectroscopy comparison before oxidation and after oxide removal, in order to have comparison between WSe2of same thickness. No apparent change in peak position is observed, implying no crystalline damage due to plasma oxidation.cX-ray photoelectron spectroscopy (XPS) comparison of as flaked WSe2and plasma-oxidized WSe2. The appearance of two additional peaks after oxidation corresponds to anxfactor of 3 in WOx.dW 4f core level XPS spectrum comparison of pristine WSe2and plasma-oxidized WSe2. The observed shift to lower binding energy implies electron transfer from WSe2to WO3 More importantly, the potential of such nanomaterials for low-temperature, large-area transfer and integration, independent of their material synthesis [5] , [6] , puts them in an advantageous position to be co-integrated additively with metal interconnects on CMOS (complementary metal–oxide–semiconductor) chips (Supplementary Table 1 ). The feasibility of 3D integration with CNTs has already been demonstrated by Shulaker et al. [1] , but that of 2DMat has only started to gain traction [7] . 2DMat, with their intrinsic nanolayer structures and variety of electronic structures are expected to add more functionalities for process temperature-limited technologies like sequential/monolithic 3D chips [8] and high-performance flexible electronics [9] . In this work, we demonstrate the feasibility of hybrid co-integration of a surface-engineered WSe 2 -based thin film transistor (TFT) and resistive random access memories (ReRAM) to realize a 1 transistor–1 resistor (1T1R) memory cell. This is done through integrating WSe 2 of different morphologies (single crystalline for TFT, and polycrystalline for ReRAM) processed through different synthesis technique, to address the conflicting charge transport attributes required for logic and memory. As TFT should be optimized for high performance and low leakage, the high-quality mechanically exfoliated WSe 2 is utilized as the transistor channel. On the other hand, ReRAM should be optimized for low-voltage defect-enabled switch ability, for which solution-processed WSe 2 is employed. Despite WSe 2 2DMat being well investigated for future logic application, its application for 1T1R memory cell by hybrid co-integration is yet to be investigated. Moreover, our proposed processes are room temperature based, offering compelling compatibility with temperature-limited 3D monolithic process integration and flexible electronics processing. Furthermore, we propose through calibrated compact device modeling and circuit simulations that sub-0.01 µm 2 1T1R cells with good read/write margins are feasible by stacking 2D nanosheets to realize a multiple-stacked 2D TFTs to drive the 2D ReRAMs. WSe 2 select transistor material With a large bandgap, a reasonably high intrinsic thin-channel carrier mobility [10] , and n – p polarity that can be easily modulated by contact Schottky barrier metal [11] , WSe 2 offers great potential for low leakage and performant CMOS logic gates [12] . The low on-state resistance and off-state leakage potential of the WSe 2 transistor also makes them a good select transistor candidate for 1T1R memories, which calls for minimization of voltage loss across the transistor during memory cell set/reset and the off-state sneak current in the array, respectively. Despite the favorable intrinsic attributes, WSe 2 transistors are still challenged by extrinsic degradations in mobility and high contact resistance. The reports of WSe 2 exhibiting high mobility at low temperatures [13] suggest the detrimental role played by various scattering sources, such as phonons, Coulomb impurities (CI), and intrinsic defects in mobility degradation. Although passivation methods based on dielectric deposition, including atomic layer-deposited high- k encapsulation [14] , have been pursued, the process uniformity remains challenging due to undesired grain boundary nucleation [15] . Thus, it becomes necessary to investigate other strategies including uniform native oxide passivation solution as well. In addition, minimizing transistor access resistance is essential to translate the performance gains from channel carrier mobility. While heavy source/drain (S/D) doping is the most preferred method for improving contact resistance in conventional Si devices, such substitutional doping in 2DMat comes at the expense of increased defect density [16] . For 2DMat, several approaches ranging from material modification to the co-integration of graphene electrodes [17] have been proposed. However, they present new challenges in stability and work-function limitations. For example, the semiconducting 2H phase to metallic 1T phase modification [18] can improve contact resistance significantly, but the low-temperature stability and Fermi level to conduction band alignment limits its utilization for p -FETs [14] . Graphene contacts, due to its Fermi level alignment close to the conduction band, would also lead to undesirable electron injection for p -FETs [17] . In this work, we concurrently address strategies for hole carrier doping, mobility enhancement, Schottky barrier, and contact resistance reduction through a single-step process that overcomes the issues of stability and p -contact work-function alignment. We developed a self-limiting single-step, low-temperature WO 3 formation on channel surface and under the S/D contacts by post-contact remote plasma oxidation. This process simultaneously enhances the WSe 2 TFT mobility by almost 76 times and reduces the contact resistance by a hundred-fold. By implementing Ag-WO 3 -WSe 2 metal–insulator–semiconductor (MIS) contact, we achieved an ultra-low Schottky barrier height (SBH) of 25 meV with respect to the WSe 2 valence band, significantly enhancing hole injection. Low-temperature surface layer plasma oxidation for WSe 2 FET For 2D transition metal dichalcogenides (TMDs), the thickness is a critical parameter influencing their electronic and optical properties. Although mechanical exfoliation results in high-quality WSe 2 flakes, the approach does not allow for precise thickness control. Considerable amount of research has been devoted to realizing a thickness reduction strategy, such as the use of focused ion beam [19] , ozone treatment [20] , [21] , XeF 2 vapors [22] , plasma oxidation [23] , thermal oxidation [24] , and so on. However, these approaches can induce minor [22] as well as major damage to the crystallinity of the WSe 2 material with resultant negative impact to its electrical performance. While the above-mentioned reports focus on oxidation as a thickness reduction strategy for mechanically exfoliated samples, we introduce a low-temperature remote plasma oxidation process (Methods section) and study the utility of the formed oxide as a MIS contact and encapsulation layer using detailed material and electrical characterization. We show that gentle plasma oxidation can create a layer of surface WO x , which do not damage the underlying WSe 2 structure. Figure 1a shows the cross-sectional transmission electron microscope (xTEM) image of the WSe 2 flake before and after the remote plasma oxidation, from which the presence of WO x and the quality of exposed WSe 2 are confirmed. The thickness of the formed WO x is ~2.2 nm for a consumption of three layers of WSe 2 , as confirmed by xTEM. Irrespective of oxidation time, the WO x formation is found to be self-limiting as well (Supplementary Fig. 1 ). The same oxide thickness has been validated for WSe 2 of different starting area and thicknesses under the same oxidation condition. Fig. 1 Remote plasma oxidation process and characterization. a Schematic representation of surface plasma oxidation and the corresponding cross-sectional transmission electron microscope (xTEM) images. The xTEM image of oxidized WSe 2 shows 2.2 nm of WO 3 upon oxidation, which is a consumption of three layers of WSe 2 . b Raman spectroscopy comparison before oxidation and after oxide removal, in order to have comparison between WSe 2 of same thickness. No apparent change in peak position is observed, implying no crystalline damage due to plasma oxidation. c X-ray photoelectron spectroscopy (XPS) comparison of as flaked WSe 2 and plasma-oxidized WSe 2 . The appearance of two additional peaks after oxidation corresponds to an x factor of 3 in WO x . d W 4f core level XPS spectrum comparison of pristine WSe 2 and plasma-oxidized WSe 2 . The observed shift to lower binding energy implies electron transfer from WSe 2 to WO 3 Full size image Raman spectroscopy and X-ray photoelectron spectroscopy (XPS) analysis were done to determine the nature of WO x formed by this process. As the vibrational and optical properties strongly vary with thickness, a comparison of “oxidized WSe 2 ” and “oxide-removed WSe 2 ” has been performed. The oxide removal process, which is selective to WSe 2 , is done using KOH solution (Methods section). From the Raman spectrum in Fig. 1b , we observe the typical out-of-plane A 1g mode, in plane E 2g mode and the bulk, B 2g mode for two prepared four-layer WSe 2 samples; one with WO x (after oxidation) and one without WO x (after oxide removal). No apparent Raman peak shift is detected between the two samples—ruling out the presence of any plasma oxidation induced stress in WSe 2 . The resultant WO x appears to be amorphous due to the absence of the 800 cm −1 signature peak, indicating crystalline WO x [25] (Supplementary Fig. 2 ). The amorphous WO x structure is further corroborated by the xTEM images (Fig. 1a ), which did not reveal any crystalline order in the WO x layer. Since there exists reports of crystalline WO 3 formed through air heating at higher temperature of 400 °C [25] , the amorphous WO x is likely due to our low-temperature plasma oxidation process. From the XPS analysis in Fig. 1c , we confirm the stoichiometry of amorphous WO x to be native WO 3 . Specifically, peaks at 35.5 and 37.7 eV after plasma oxidation correspond to the binding energies of W 6+ , indicating the presence of WO 3 [25] . Furthermore, we observe charge transfer mediated by WO 3 from the XPS spectrum after plasma oxidation. The observed decrease in binding energy of W 4f core levels (0.18 eV reduction in W 4+ 4f 7/2 and 0.26 eV reduction in W 4+ 4f 5/2 ) (Fig. 1d ) suggests that there is electron transfer from WSe 2 to WO 3 . This is attributed to the high work function of WO 3 consistent with other reported studies [22] . We show here that low-temperature plasma oxidation, capable of self-limiting to ~2.2 nm amorphous WO 3 , produces an ultra-thin hole donor layer that is also gentle to WSe 2 . 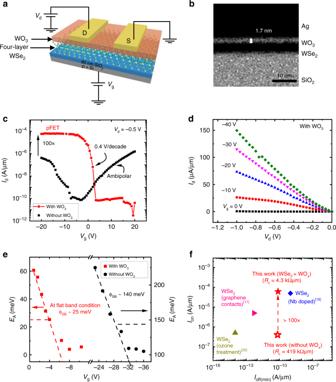Fig. 2 Surface plasma-oxidized WSe2TFT and electrical characterization.aDevice schematic showing a four-layer WSe2and 2.2 nm WO3on SiO2/p+ Si layer with gate length (Lg) = 1.80 µm and width (W) = 2.05 µm.bTransmission electron microscopy image of the device contact region, after post-contact plasma oxidation, revealing the presence of WO3underneath the metal contacts. cId–Vgplots for four-layer thick device with and without WO3.dId–Vdcharacteristics after plasma oxidation for different gate voltages.eEffective Schottky barrier height extraction from low-temperature transfer characteristics and Arrhenius plot. At flat band condition, the curve deviates from linearity and the corresponding activation energy becomes the Schottky barrier.fBenchmark plot showing the performance of plasma-oxidizedp-FET versus other reported data.Ionis determined atVd= −0.5 V Figure 2a shows the schematic of the fabricated device consisting of a four-layer WSe 2 and three-layer WO 3 . The detailed fabrication procedure can be found in the Methods section. In order to realize a thinner WO 3 layer under the Ag S/D contacts to minimize tunneling resistance, we chose to perform post-contact plasma oxidation. The key advantage of this strategy is that the WO 3 growth rate under the S/D region would be moderated by the metal contact. The TEM image (Fig. 2b ) confirms thinner (1.7 nm) WO 3 layer under the contact as opposed to the thicker (2.2 nm) oxide formation for the exposed channel, despite the common plasma oxidation process. Due to limited diffusion of O radicals at the Ag-WSe 2 terminations on both ends of the electrodes, the O radicals can only propagate laterally under the Ag contacts, resulting in a reduced thinning of WSe 2 layer [24] under the contact metal as opposed to the exposed channel regions. Fig. 2 Surface plasma-oxidized WSe 2 TFT and electrical characterization. a Device schematic showing a four-layer WSe 2 and 2.2 nm WO 3 on SiO 2 / p + Si layer with gate length ( L g ) = 1.80 µm and width ( W ) = 2.05 µm. b Transmission electron microscopy image of the device contact region, after post-contact plasma oxidation, revealing the presence of WO 3 underneath the metal contacts . c I d –V g plots for four-layer thick device with and without WO 3 . d I d –V d characteristics after plasma oxidation for different gate voltages. e Effective Schottky barrier height extraction from low-temperature transfer characteristics and Arrhenius plot. At flat band condition, the curve deviates from linearity and the corresponding activation energy becomes the Schottky barrier. f Benchmark plot showing the performance of plasma-oxidized p -FET versus other reported data. I on is determined at V d = −0.5 V Full size image We characterized the resultant TFT performance by measuring the transfer and output characteristics (Fig. 2c, d ). Figure 2c compares the transfer characteristics with and without post-contact plasma oxidation. The devices without WO 3 is unremarkable, showing ambipolar conduction, with slightly stronger n-type ( V g >−5 V) than p -type conduction ( V g <−5 V). Upon plasma oxidation, the device exhibits strong p - type conduction. Most remarkably, a 100× enhancement in the hole current is accompanied by a strong polarity change, where n-type conduction is completely suppressed. To further investigate the TFT performance improvement, we carefully characterized the influence of WO 3 on mobility and contact resistance. We measured the gate inversion capacitance of the oxidized device and found it to have increased by 2× compared to the geometrical value (77 vs. 38 nF cm −2 ). Details of inversion capacitance extraction are found in Supplementary Fig. 3 and Supplementary Note 1 . 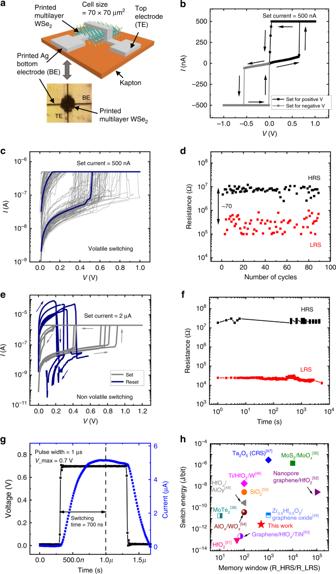Fig. 3 Printed WSe2ReRAM electrical characterization.aSchematic of printed WSe2ReRAM with Ag contacts along with microscope image of printed ReRAM.bThe device sets from HRS to LRS for both positive and negative voltages.cStress cycling data for 90 cycles at a smaller set current of 500 nA, where volatile behavior is observed.dEndurance properties of ReRAM at read voltage of 50 mV and a set current of 500 nA.eSet and reset operation with a larger set current of 2 µA, exhibiting non-volatile behavior.fRetention plot showing LRS and HRS stability till 104s at a read voltage of 50 mV and set current of 5 µA.gSwitching time characterization with an AC pulse of 0.7 V amplitude and 1 µs pulse width.hBenchmark plot of switching energy per bit vs. memory window of printed WSe2ReRAM with other representative non-volatile resistive switching publications Since we do not observe CV frequency dispersion (Supplementary Figure 3e ) that indicates significant fast or slow charge trapping/de-trapping processes, we exclude the possibility of spurious charges and disorder at WSe 2 bottom-gate dielectric interface as reported by Pradhan et al. [13] . Instead, we believe the interfacial charge transfer at the WSe 2 -WO 3 heterostructure contributed towards the capacitance increase. To ensure accurate mobility extraction, we emphasize here the need for CV measurements, instead of making capacitance assumptions based on geometry. From Fig. 2c and the measured inversion capacitance, we extracted a dramatic 76× hole field-effect mobility ( µ FE ) increase from 3 cm 2 V −1 s −1 (non-oxidized) to 230 cm 2 V −1 s −1 and observed a significant 100× reduction of contact resistance ( R c ) to 4.3 kΩµm from our control with 420 kΩµm, which is extracted using the well-reported R total –V g method [26] . The details of field-effect mobility and contact resistance extraction can be found in the Supplementary information (Supplementary Figs. 4 and 5 ). The R c reduction correlates to a considerable lowering of the contact’s SBH to 25 meV with respect to the SBH of 140 meV of our control sample without WO 3 as shown in Fig. 2e . It appears that the thin WO 3 under the Ag contact unpinned the contact Fermi level with respect to WSe 2 , closer to the valence band minimum of WSe 2 , owing to the high work function of WO 3 [27] . This would also explain the observed suppression of electron current, as the SBH for electrons would be large. Our room temperature, low-power remote plasma oxidation treatment allows a gentler process to achieve less damage to the underlying WSe 2 flake, as evident by the non-reduction of the PL signal [23] (Supplementary Fig. 6 ) as compared to other reported methods [28] . In addition, the plasma process allows the formation of a uniform thin layer of WO 3 beneath the contact, which has not been reported. The argument is supported by the observed SBH to be 10× lower than the barrier height reported from other work involving similar surface functionalization with WO 3 [20] . Furthermore, we conducted an experiment, where the plasma oxidation was performed prior to contact formation, leading to a uniform thicker (2.2 nm) WO 3 under S/D contacts and over the channel (Supplementary Fig. 7 ). While the drive current slightly improved compared to non-oxidized device, the performance is weaker than the post-contact-oxidized sample due to higher contact resistance, which is comparable to the device without oxidation (Supplementary Fig. 5 ). This suggests the importance of controlling WO 3 thickness, as a tunneling layer—the thicker WO 3 with pre-contact oxidation actually degrades the contact resistance due to increased tunneling resistance [29] . Figure 2f benchmarks selected top-performing WSe 2 devices from various reports. Our work shows the strongest I on performance for devices with sub-nA µm −1 -level I off_min , showing an extraordinary 100× drive current enhancement with respect to our non-WO 3 control (Supplementary Table 2 ). WSe 2 ReRAM material, fabrication, and characterization 2DMat-based ReRAM on multilayer hBN [30] , [31] , solution-processed multilayer 2D ReRAM [32] , [33] , [34] , [35] , MoS 2 phase change memristor behavior [36] , novel resistive switching approaches such as gate tunable non-volatile resistive switching in monolayer MoS 2 via atomic re-arrangement of grain boundaries [37] , and fast switching operation enabled by electric field-induced structural transition in MoTe 2 and Mo 1 − x W x Te 2 [38] have been demonstrated. Here, we investigate the potential of a Ag-WSe 2 -Ag ReRAM comprising of a solution-processed WSe 2 as the resistive memory element and Ag as electrodes, realized using a high-precision Aerosol Jet printing (Methods section and Supplementary Table 3 ). Apart from being compatible with 3D monolithic integration, the solution-processed approach combined with the aerosol jet printing is chosen to leverage on the in situ sonication-induced modulation of defects in the switching layer through ink quality to study the device impact due to different WSe 2 morphologies [39] . Compared to traditional metal oxide-based ReRAMs, the realization of forming-free operation with lower switching voltage and current is one of the defining advantages of solution-processed WSe 2 ReRAM. This may be due to the defect formation and migration with respect to the flake morphology as opposed to shorted metallic conductive bridges in oxide ReRAM [40] . Together with the unique material properties, we demonstrate Ag/WSe 2 /Ag ReRAM that exhibits non-volatile, forming-free, sub-1 V switching characteristics at a set current ≤5 µA, with a low switching energy of 2.9 pJ per bit. Figure 3a shows the schematic and the optical microscope image of the WSe 2 ReRAM with Ag contact. We performed a detailed material characterization using scanning electron microscopy (SEM), Raman spectroscopy and X-ray diffraction (Supplementary Fig. 8 ). As observed from SEM images, the morphology of the as-printed WSe 2 layer is highly disordered with randomly distributed clusters, significantly different from the exfoliated-transferred WSe 2 for the TFT. Raman analysis shows that the E 2g mode of the printed WSe 2 is consistent with the exfoliated WSe 2 . The absence of interlayer coupling-B 2g mode and the out-of-plane A 1g mode is likely due to the disordered morphology of the printed WSe 2 . The non-orientated switching layer morphology is desired for the vertical memory element as we seek to promote volume-based vacancy or filamentary switching for our devices. Figure 3b shows the direct current (DC) sweep characteristics over a voltage range of −1 to 1 V with a set current limit to 500 nA. The device exhibits forming-free behavior, which can be set in both positive and negative polarity bias. We observe an abrupt switching at sub-1 V set voltage, indicating filamentary-based conduction. Under a set current of 500 nA, the switching characteristic is found to be volatile, that is, the low resistance state (LRS) decays quickly to high resistance state (HRS) after the bias is removed. Figure 3c shows the DC stress cycling of the device over 90 cycles, while Fig. 3d shows the repeatability of the HRS/LRS over the 90 cycles at a read voltage of 50 mV. The device achieves an average HRS/LRS window of ~70 over all the cycles tested. When the set current is increased to 2 µA, the device transitions to a non-volatile switching state. We believe that with the larger set current, the filament thickens and remains stable without external bias [41] . The ReRAM exhibits a unipolar switching behavior where set and reset voltages share the same polarity. As observed in many of the unipolar ReRAM, the reset operation is dominated by the thermophoresis effect [42] , where joule heating ruptures the filament, thus returning the device to the HRS state. The reset voltage ranges from 0.2 to 0.3 V, while the reset current lies in between 80 and 100 μA, as shown in Fig. 3e . The observation of the unipolar switching characteristics is concomitant with that of chemical vapor deposition-grown WSe 2 reported by Ge et al [43] . We observe a larger memory window of 10 3 when the set current is increased to 5 µA and achieves a retention time of >10 4 s (Fig. 3f ). Fig. 3 Printed WSe 2 ReRAM electrical characterization. a Schematic of printed WSe 2 ReRAM with Ag contacts along with microscope image of printed ReRAM. b The device sets from HRS to LRS for both positive and negative voltages. c Stress cycling data for 90 cycles at a smaller set current of 500 nA, where volatile behavior is observed. d Endurance properties of ReRAM at read voltage of 50 mV and a set current of 500 nA. e Set and reset operation with a larger set current of 2 µA, exhibiting non-volatile behavior. f Retention plot showing LRS and HRS stability till 10 4 s at a read voltage of 50 mV and set current of 5 µA. g Switching time characterization with an AC pulse of 0.7 V amplitude and 1 µs pulse width. h Benchmark plot of switching energy per bit vs. memory window of printed WSe 2 ReRAM with other representative non-volatile resistive switching publications Full size image We have confirmed that the switching is not due to Ag ion diffusion in WSe 2 by comparing the ReRAM switching behavior of otherwise identical devices with inert carbon-based electrodes (Supplementary Fig. 9 and Supplementary Discussion 1 ), which show similar abrupt switching characteristics. This indicates that the switching mechanism is intrinsic to the WSe 2 switching layer, likely due to selenium vacancies, thus ruling out the possibility of Ag metal ion conductive-bridge-based mechanism. The switching time, as calculated by applying a voltage pulse of amplitude 0.7 V and 1 μs width is found to be 700 ns (Fig. 3g ). With the trade-off existing between programing voltage and switching time [44] , we have chosen to limit the programming voltage to achieve low set power, which results in slower switching time of 700 ns. From the material/structural point of view, controlling the flake size and thickness of the switching layer would be areas that could potentially offer improvement in switching speed [45] . Our devices show one of the lowest reported switching energy (Supplementary Fig. 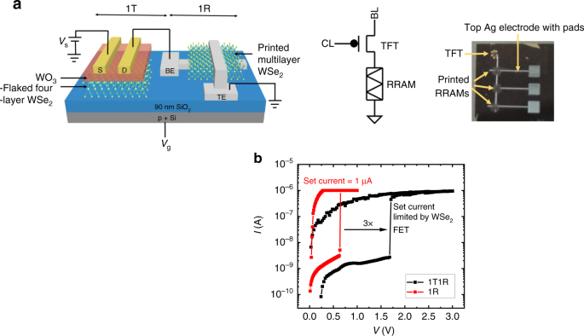Fig. 4 1T1R configuration and characterization.a3D schematic view of 1T1R structure with flaked WSe2transistor and printed WSe2ReRAM and the corresponding circuit representation. The photo image of 3× WSe2ReRAMs printed using low-temperature aerosol jet printing method, which is linked up to the fabricated WSe2TFT on a single chip is also shown.bI–Vswitching plot for 1T1R configuration, where the switching current is limited by the transistor drive current 10 , Supplementary Table 4 , and Supplementary Note 2 ) relative to other 2DMat [35] , [38] and other oxide-based ReRAMs [46] , [47] , [48] , [49] , [50] , [51] , [52] , [53] , [54] , as illustrated in the Fig. 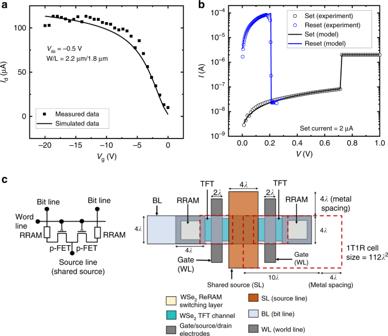Fig. 5 Compact modeling and circuit simulations.aId–Vgof SPICE TFT model vs. measured WSe2p-FET.bI–Vof SPICE ReRAM model vs. measured for SET and RESET process.cCircuit representation and layout of shared SL 1T1R structure, with the 1T1R cell size indicated (BL—bit line; WL—word line; SL—shared-source line) 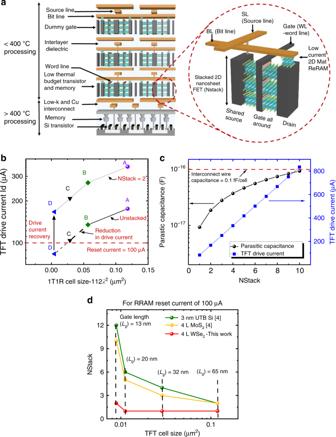Fig. 6 3D monolithic stacking of TFT and memory.aConceptual illustration of 3D monolithic stacking of CMOS logic and 2D multiple-stacked WSe2TFTs with ReRAM with thermal budget indicated for various levels (not to scale).bTransistor drive current (atVsg= 2 V) variation with respect to 1T1R cell size as perλdesign rule. The specifications for the legends are, A:Lg=65 nm, Wch=130 nm, EOT = 2.3 nm,k= 4.5;B:Lg= 45 nm,Wch= 90 nm, EOT = 2.2 nm,k= 4.5; C:Lg= 32 nm,Wch= 64 nm, EOT = 2.1 nm,k= 4.5; D:Lg= 13 nm,Wch= 26 nm, EOT = 1.1 nm,k= 25. We observe ~2.25× drop in drive current as the width is scaled 5× (130–26 nm). Stacked-channel devices showing the recovery of drain current with NStack = 2, to support the ReRAM reset current of 100 µA.cChange in TFT drive current and parasitic capacitance (self-capacitance due to stacking) vs. NStack (number of 2DMat nanosheet stacking layer) atVsg= 2 V.dComparison of NStack (number of nanosheet TFT stacked) for different feature sizes among WSe2, MoS2, and UTB Si to support ReRAM reset current of 100 µA 3h with endurance comparable to other reported 2DMat ReRAMs (Supplementary Table 5 ). We suspect that the low switching energy is promoted by the excess defects and grain boundaries in our printed WSe 2 layer. We performed repeatability check for ReRAM devices fabricated across several batches at different times, where we observed consistent switching characteristics, as shown in the cumulative probability distribution plot for set voltage, reset voltage, and ReRAM resistance (Supplementary Fig. 11 ). We believe that there is still significant opportunity for improvement with respect to ReRAM endurance and other metrics by engineering the flake sizes with the solution-processed approach. Although Aerosol jet printing technique allows additive deposition of inks with a wide range of viscosities to realize quick prototyping of devices at relaxed dimensions (down to 10 μm feature size), it is not a suitable method for industrial-scale production because of the low throughput and large feature size achievable. Except for the low thermal budget of our process, we do not believe that our additive approach would significantly change the device conclusions for the solution-deposited and subtractive methods like solution spin coating, compatible with large-scale dense circuit integration. All WSe 2 1T1R memory cell integration and characterization The approaches of in-memory and neuromorphic computing based on embedded memory have recently garnered great momentum, with growing interests to apply ReRAM [55] . However, high-density cross-bar ReRAM array suffers from current cross-talk interference due to sneak currents [56] , resulting in misreading and unintended disturbance of memory states as well as undesirable increase in memory standby power consumption. By employing a select transistor to isolate the selected ReRAM cell from unselected cells, a 1T1R architecture can be implemented to circumvent these problems [57] , [58] . Since the 1T1R cell leakage is gated by the select transistor off-state leakage, it is necessary for the select transistor bandgap to be appropriately wide to limit S/D band-to-band leakage current due to the memory operating voltage. WSe 2 possess suitable bandgap in the range of 1.2 eV (bulk) to 1.6 eV (monolayer), limiting the transistor minimum off-state leakage to be in the order of pA μm −1 for operating voltages in the range of 0.8–1.5 V. On the other hand, the maximum on-state drive current of the select transistor should support the set voltage and reset current of the ReRAM. However, the low intrinsic drive current of 2D TMD-based TFT makes it difficult to drive the ReRAM. Therefore, we propose to utilize the performance enhancement in plasma-oxidized WSe 2 to mitigate this issue. We integrated the TFT and the ReRAM on the same chip to study the co-integration and its functionality (Fig. 4a ), where the WSe 2 ReRAM is printed after the WSe 2 TFT fabrication. The measured 1T1R circuit configuration is as depicted in Fig. 4a . Figure 4b shows the successful switching of the WSe 2 ReRAM by the WSe 2 TFT. As expected, the TFT’s on-state resistance increased the memory cell switching voltage to 1.7 V, which is almost 3× larger than that of the ReRAM alone. This clearly highlights the gating impact of the select transistor performance for the memory cell. It is necessary to decrease the TFT on-state resistance while maintaining low off-state leakage to limit sneak current. This becomes increasingly challenging with decreasing cell size where TFT area is constrained. In the next section, we investigate the cell design with the use of material-calibrated compact models and circuit simulations, which would allow us to project for scaled-up memory array implementation. Fig. 4 1T1R configuration and characterization. a 3D schematic view of 1T1R structure with flaked WSe 2 transistor and printed WSe 2 ReRAM and the corresponding circuit representation. The photo image of 3× WSe 2 ReRAMs printed using low-temperature aerosol jet printing method, which is linked up to the fabricated WSe 2 TFT on a single chip is also shown. b I – V switching plot for 1T1R configuration, where the switching current is limited by the transistor drive current Full size image Material-device-circuit co-design of 1T1R memory cell In order to evaluate the memory cell for scaled technologies and to project for future 1T1R technology, we investigate the material-system co-design using detailed circuit modeling and study the disruptive impact of material properties on the system design considerations. A BSIM-IMG compact circuit model [59] description of the TFT has been calibrated to experiment-based long-channel devices and known WSe 2 material parameters. Short-channel effects such as velocity saturation, GISL (gate-induced source leakage) and GIDL (gate-induced drain leakage) has been taken into account for the scaled devices through modeling. A hysteron-based compact model, as reported by Garcia-Redondo et al. [60] , has been calibrated to the WSe 2 ReRAM. Guided by experimental data, we applied these models largely behaviorally, given that the physics of these devices are not well described yet. Despite this, we expect these models to be accurate for our SPICE circuit analysis. Figure 5a, b show the compact model behavior for WSe 2 TFT and ReRAM, respectively, which correlates well with the experimental data. Fig. 5 Compact modeling and circuit simulations. a I d –V g of SPICE TFT model vs. measured WSe 2 p -FET. b I – V of SPICE ReRAM model vs. measured for SET and RESET process. c Circuit representation and layout of shared SL 1T1R structure, with the 1T1R cell size indicated (BL—bit line; WL—word line; SL—shared-source line) Full size image We project scaled technology performance by calibrating our device and circuit models with intrinsic long-channel mobility and contact resistance enhancement salient to our 2D WSe 2 approach. Our aim is to provide a first-order comparison between different material systems and their potential system impact, without the distraction of subjective details specific to scaled device design (such as interface trap density, S/D tunneling, etc. as explained in Supplementary Fig. 12 and Supplementary Discussion 2 ) and other more complex technology factors. We recognize that detailed technology factors related to scaled transistor/memory device behavior, interconnect properties, physical layout, and process integration approaches would be useful to refine the system view in the future. Here, we analyze the 1T1R cell scaling using λ -based design rule description, where F = 4 λ = minimum metal ½ pitch and 1T1R cell size is limited by the select transistor size (min. cell area = 112 λ 2 ) [61] . The layout of such a shared-source 1T1R cell is shown in Fig. 5c . As the 1T1R memory cell is scaled down, the selector drive current degrades with the linear reduction of width ( W = 4λ ), whereas the ReRAM switching current is largely insensitive to the cell size due to filamentary switching [43] . This would raise concern over the ability of the select transistor to set and reset the ReRAM, for smaller cells. For shorter channel length, as the drive current scales with width ( W ) and C ox as per the relation, I sd,sat = V sat WC ox ( V sg − | V tp | − V sd,sat ), increasing TFT gate capacitance ( C ox ), with thinner high- k gate dielectrics (to increase carrier charge density) may compensate for the current degradation due to width scaling [62] . However, our analysis shows that, even with aggressive scaling of high- k gate oxide as per industry standards for low-power devices [62] , [63] , we would still suffer a 2.2× drop in current as the width is reduced 5× (from gate length of 65 to 13 nm in Fig. 6b ). Fig. 6 3D monolithic stacking of TFT and memory. a Conceptual illustration of 3D monolithic stacking of CMOS logic and 2D multiple-stacked WSe 2 TFTs with ReRAM with thermal budget indicated for various levels (not to scale). b Transistor drive current (at V sg = 2 V) variation with respect to 1T1R cell size as per λ design rule. The specifications for the legends are, A: L g = 65 nm , W ch = 130 nm, EOT = 2.3 nm, k = 4.5 ; B: L g = 45 nm, W ch = 90 nm, EOT = 2.2 nm, k = 4.5; C: L g = 32 nm, W ch = 64 nm, EOT = 2.1 nm, k = 4.5; D: L g = 13 nm, W ch = 26 nm, EOT = 1.1 nm, k = 25. We observe ~2.25× drop in drive current as the width is scaled 5× (130–26 nm). Stacked-channel devices showing the recovery of drain current with NStack = 2, to support the ReRAM reset current of 100 µA. c Change in TFT drive current and parasitic capacitance (self-capacitance due to stacking) vs. NStack (number of 2DMat nanosheet stacking layer) at V sg = 2 V. d Comparison of NStack (number of nanosheet TFT stacked) for different feature sizes among WSe 2 , MoS 2 , and UTB Si to support ReRAM reset current of 100 µA Full size image One way to address the issue of weak select transistor would be to rely on smaller ReRAM set current, but at the expense of reduced HRS/LRS ratio (Supplementary Fig. 13 ). Hence, to mitigate the drive current degradation, without compromising on the memory window, we propose increasing the effective width by vertical stacking of 2DMat nanosheet TFT channels. This would allow for TFT drive current recovery, without sacrificing the 1T1R cell footprint. The conceptual representation of such a 3D monolithic stacking of CMOS logic and 2D multiple-stacked WSe 2 TFTs is shown in Fig. 6a . While thin WO 3 is still utilized as hole doping layer, an additional gate dielectric with a metal gate wrapped around the nanosheet could be employed, to realize the proposed gate all around (GAA) vertically stacked WSe 2 TFT. Accordingly, as shown in Fig. 6b , an NStack (number of 2DMat nanosheet TFT channels) of 2 would more than compensate for the drive current loss due to geometric width scaling, to support ReRAM reset current of 100 µA. Although stacking of channel layers would result in boosted drive current per footprint, the parasitic capacitance arising from the self-capacitance due to stacking including gate to S/D capacitance and other fringing components could lead to increased switching delays and slowing down of circuit operation. Hence, it is necessary to evaluate the trade-off between the number of stacking layers and the cell switching delay due to transistor capacitance vs. wiring interconnect parasitic. The increase in parasitic capacitance with the number of stacking layers for L g = 13 nm is shown in Fig. 6c . With a metal wire pitch of 52 nm and assuming aspect ratio to be 2, the capacitance of the wire is 1.045 fF µm −1 [64] . Accordingly, the interconnect capacitance for a 1T1R cell, considering the metal line length to be 14 λ , is 0.1 fF per cell. The simulated transistor parasitic capacitance due to stacking reveals that the interconnect capacitance induced by long word line/bit line would be the more dominant factor and that the stacking-induced self-capacitance is not expected to pose a serious concern for NStack ≤10. The necessity for having a high performant stacking channel layer becomes even more critical, to restrict the NStack below 10. With GAA nanosheet FETs being regarded as a potential candidate for sub-3 nm technology node, the key research areas that require improvements are fine-tuning of nanosheet width optimization with extreme ultraviolet lithography [65] , optimization of inner spacers [66] , advancement in metrology, and inspection to measure the buried channel, process control, and other fabrication challenges in gate stack integration. Furthermore, we have compared the number of stacking layers that would be required for other 2D materials such as MoS 2 as well as conventional ultrathin Si from other reported works with respect to the WSe 2 device reported in this work. Our analysis shows that the enhanced WSe 2 device requires a fewer number of channel stacking layers as compared to other materials, to support the maximum reset current of 100 µA of our low-voltage ReRAM (Fig. 6d ). This is due to WSe 2 ’s higher mobility at sub-5 nm channel thickness, compared to MoS 2 and ultrathin Si. Specifically, only two 2D WSe 2 TFT channel stacks (NStack = 2) are required for cell sizes below 0.01 µm 2 . These findings imply that, apart from thermal budget limitation, the large number of stacking layers required for ultrathin Si transistors and MoS 2 at sub-5 nm channel thickness increases the complexity of fabrication and the stacking-induced parasitic capacitance. While smaller effective mass ( m* ) of WSe 2 allows for higher mobility and high performance in sub-10 nm gate length ( L g ), the enhanced S/D tunneling due to lower m* is the down side [67] , [68] . Hence, to further reduce the footprint of each device, we recommend greater width scaling rather than L g scaling, without increasing the standby power. However, the width scaling will come at the expense of lower drive current per TFT. In this case, channel stacking of TFT becomes even more necessary to recover the required drive current and is an essential control knob to enable dense 1T1R cell. In this work, a low-thermal-budget hybrid (solution-processed-exfoliated) integration of 2D material-based 1T1R is demonstrated for the first time. We highlight the importance of different material morphology for logic and memory operation. The select transistor needs to be single crystalline with enhanced drive for scaled 1T1R cells, while it is desired for the memory device to be polycrystalline with defects that enable low-voltage switching. We show by post-contact plasma oxidation, a simple low-thermal-budget method to enhance the multilayer WSe 2 transistor for this purpose; achieving significant hole mobility (230 cm 2 V −1 s −1 ), reduction of contact resistance (to 4.3 kΩµm) and Schottky barrier (to 25 meV). This culminates in a 100× drive enhancement with respect to our control devices. In addition, we report an all-printed WSe 2 -based ReRAM using a low-temperature, aerosol jet process. The ReRAM exhibits sub-1 V non-volatile unipolar switching with a low switching energy of 2.9 pJ per bit. We demonstrated the TFT-ReRAM 1T1R hybrid co-integration, which guided our accurate device-circuit models and enabled us to investigate material-system memory cell co-design for scaled technologies. This led us to the proposed stacked TFT channels for the memory cell to achieve high-density 1T1R memory array for future dense monolithic 3D memory systems. Methods Remote plasma oxidation The plasma chamber source to sample distance is limited to 10 cm. The oxidation is performed at room temperature with a plasma power of 11 W and chamber pressure of 20 mTorr (100 sccm of O 2 and 20 sccm of Ar) for 2 min to form 2.2 nm WO 3 . For some of the material characterization, the WO 3 is removed by dipping in 1 M KOH solution for 30 s. TFT device fabrication and characterization WSe 2 flakes were mechanically exfoliated on p + Si with 90 nm SiO 2 layer, followed by electrode patterning using electron beam lithography. The length and width of the device are characterized and validated by AFM. Ag (10 nm) contacts capped with Au (90 nm) was deposited by electron beam evaporator followed by lift off to form source and drain contacts. The device is then subjected to an annealing procedure (200 °C for 1 h in N 2 -H 2 ambient, followed by vacuum annealing at 250 °C for 0.5 h), to remove the photoresist residue and other gaseous adsorbates. After which, the plasma oxidation, as explained in the previous step is performed to form WO 3 above the channel and also underneath the S/D contacts. The electrical measurements were collected by Agilent parameter analyzer B1500A. Aerosol ink printing method for WSe 2 ReRAM WSe 2 flakes suspended in ethanol forms the ink (concentration 0.1 mg/ml, from 2D semiconductor) that is ultrasonically atomized and deposited by the Optomec AJ5X Aerosol Jet 5-axis Printer [69] . The bottom and top Ag electrodes are printed via the pneumatic atomizer followed by an 830 nm laser sintering process (Kapton) or a 150 °C, 30 min baking process (SiO 2 /Si substrate). Due to the low concentration of WSe 2 in the ink, the ReRAM WSe 2 layer has to be deposited over multiple passes. We deposited ~400 nm average thickness of WSe 2 (printed over 30 passes) for our ReRAM devices, with more details provided in the Supplementary Information (Supplementary Table 3 and Supplementary Fig. 8a ). A final step of baking the entire sample at a temperature of 100 °C for 30 min is done to ensure conductivity of the printed Ag electrodes.